Exploration of pyrazine-embedded antiaromatic polycyclic hydrocarbons generated by solution and on-surface azomethine ylide homocoupling 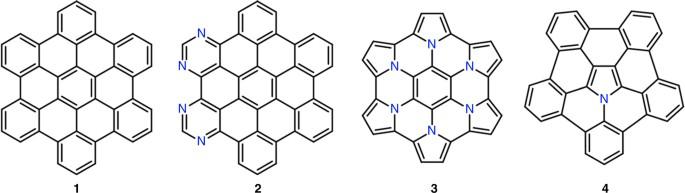Fig. 1 Chemical structures of pristine and N-doped nanographenes. Hexa-peri-hexabenzocoronene (HBC)1, periphery-doped tetraaza-HBC2, azacoronene derivatives3, and azacorannulene4 Nanographenes, namely polycyclic aromatic hydrocarbons (PAHs) with nanoscale dimensions (>1 nm), are atomically precise cutouts from graphene. They represent prime models to enhance the scope of chemical and physical properties of graphene through structural modulation and functionalization. Defined nitrogen doping in nanographenes is particularly attractive due to its potential for increasing the number of π-electrons, with the possibility of introducing localized antiaromatic ring elements. Herein we present azomethine ylide homocoupling as a strategy to afford internally nitrogen-doped, non-planar PAH in solution and planar nanographene on surfaces, with central pyrazine rings. Localized antiaromaticity of the central ring is indicated by optical absorption spectroscopy in conjunction with theoretical calculations. Our strategy opens up methods for chemically tailoring graphene and nanographenes, modified by antiaromatic dopants. Together with the advent of graphene science, an important chapter in organic chemistry has opened exploring the synthesis of extended polycyclic aromatic hydrocarbon (PAH) systems. Large PAHs, as represented by hexa- peri -hexabenzocoronene (HBC, 1 ) with π-conjugated structures extending over 1 nm, can be regarded as structurally defined, nanoscale cutouts of graphene, designated nanographene molecules [1] , [2] , [3] . Such systems can serve as platforms both for investigating the physical and chemical properties of graphene upon heteroatom-doping, as well as for the development of semiconducting materials (see Fig. 1 ). Doped nanographenes are similarly relevant for the study of aromaticity and antiaromaticity, which are fundamental concepts of organic chemistry [4] , [5] . As proposed by Hückel [6] and later by Frost and Musulin [7] , as well as Breslow [8] , π-conjugated cycles with [4n + 2] π-electrons show aromatic character with strong stabilization while cycles with [4n] π-electrons are antiaromatic and destabilized. Despite a few theoretical suggestions on local antiaromatic “defects”, or “dopants”, in graphene [9] , [10] and rapidly increasing variety of nanographene molecules, well-defined nanographene molecules with a pronounced antiaromatic ring, i.e., a local antiaromatic element, remain challenging targets to be explored. Fig. 1 Chemical structures of pristine and N-doped nanographenes. Hexa- peri -hexabenzocoronene (HBC) 1 , periphery-doped tetraaza-HBC 2 , azacoronene derivatives 3 , and azacorannulene 4 Full size image Nitrogen (N)-doped nanographenes have attracted considerable attention due to promising electronic and magnetic properties [11] offering potential applications in metal-free catalysis [12] , [13] and sensing [14] , [15] . However, the existing synthetic protocols do not allow the precise control of the doping level and heteroatom positioning. The chemical nature of nitrogen dopants (i.e., pyridinic, pyrrolic, and “graphitic” N atoms) remains largely undefined [16] , restricting the fine-tuning of the resulting properties as well as reliable structure-property relationship elucidation. In this regard, structurally well-defined N-doped nanographene molecules offer an opportunity to accurately investigate N-doping effects. Notwithstanding, N-doping of defined nanographenes has been predominantly limited to pyridinic [17] , [18] , [19] (e.g., compound 2 [20] in Fig. 1 ) and pyrrolic (e.g., compounds 3 [21] and 4 [22] , [23] ) N atoms, which only resulted in replacing benzene rings with other N-containing 6π aromatic rings, such as pyrimidines and pyrroles. To develop nanographenes with strong antiaromatic ring dopants, we consider the possibility of incorporating a pyrazine structure inside the aromatic core, which employs two “graphitic” N atoms in the framework, thus providing additional π-electrons when compared to a benzene ring. 1,4-Disubstituted pyrazine entails intriguing chemistry, expressing 8π antiaromatic (neutral), 7π non-aromatic (cationic), or 6π aromatic (dicationic) properties, depending on its oxidation state. Thus, a pyrazine ring embedded in a carbonaceous hexagonal structure serves as a localized antiaromatic ring dopant, influencing ring and perimeter currents [24] , [25] with the potential to give rise to new types of 2D materials with unconventional semiconducting properties. Here, we report in situ solution synthesis and spectroscopy of the partially fused, pyrazine-incorporated hexabenzoperylene (HBP) derivative 6a as well as on-surface synthesis of the diaza-HBC 7c with a completely embedded pyrazine core. N-doped HBP 6a features an 8π antiaromatic core structure, as documented by 1 H NMR and UV–vis absorption spectroscopy together with density functional theory (DFT) calculations. Notably, the solution chemistry of polycyclic aromatic azomethine ylides (PAMYs) [26] can be successfully adapted on the Ag(111) surface, achieving the synthesis of 7c through surface-assisted homocoupling of the dibenzo-9 a -azaphenalene (DBAP) salt 5c and concomitant cyclodehydrogenation. High-resolution scanning tunneling microscopy (STM) and frequency-modulated atomic force microscopy (FM-AFM) [27] unambiguously elucidate the chemical structure of diaza-HBC 7c . Moreover, computational modeling using DFT indicates that 7c conserves its 8π character on the Ag(111) surface. Nucleus-independent chemical shift (NICS) [28] calculations on 6a and 7c reveal high positive values at the center and 1 Å above the center of the central pyrazine rings (NICS(0) and NICS(1) values, respectively), indicative of antiaromaticity. These results demonstrate the antiaromatic nature of pyrazine-doped nanographene molecules and provide an on-surface synthesis route to N-doping nanographene materials. Solution synthesis and characterizations The synthesis of pyrazine-embedded HBP 6a (Fig. 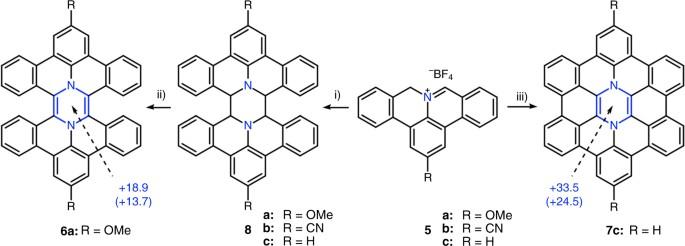Fig. 2 Synthesis of diaza-HBP6ain solution and internally N-doped diaza-HBC7cupon interfacial confinement. Reagents and conditions: (i) tributylamine, DMSO, 190 °C; (ii) DDQ, C2D2Cl4, 100 °C; (iii) in vacuo on the Ag(111) surface, 270 °C. The calculated nucleus-independent chemical shifts (NICS) values are depicted in blue (unit: ppm), indicating the antiaromatic nature of the pyrazine ring (in parenthesis the NICS(1) value, see text and Supplementary Fig.1) 2 ) was carried out based on the chemistry of DBAP, which has been employed to construct N-doped PAHs such as dibenzo[ d , k ]ullazines and 6 b 2 -azapentabenzo[ bc , ef , hi , kl , no ]corannulenes [22] , [26] , [29] , [30] . DBAP salts 5a-c with different substituents were first synthesized according to our previous method [26] . They were then dimerized to form precursors 8a–c (Fig. 2 ) by treatment with a large excess of tributylamine in dry dimethyl sulfoxide (DMSO) under argon at 190 °C. Oxidation of 8a with excess 2,3-dichloro-5,6-dicyano-1,4-benzoquinone (DDQ) in dry C 2 D 2 Cl 4 afforded diaza-HBP 6a , as characterized by 1 H NMR and mass spectroscopy (MS) analyses (Fig. 3 ). Diaza-HBP 6a turned out to be extremely unstable probably because of the antiaromatic pyrazine core, and thus the oxidation step was performed in situ in a sealed NMR tube under exclusion of air. Oxidation of other precursors 8b and 8c were also attempted with the same method, but failed to provide corresponding diaza-HBP derivatives according to 1 H NMR analysis, suggesting that the electron-donating methoxy groups of 8a played an important role in the reaction [31] . As shown in Fig. 3a , the disappearance of the characteristic signal from H F (5.13 ppm) of 8a indicated complete conversion of the starting material. All the signals in the aromatic region of 6a were down-field shifted compared to those of 8a , in agreement with the extension of the π-conjugation upon dehydrogenation. Notably, proton H E of 8a is above the neighboring benzene plane according to the optimized geometry by DFT (Fig. 4 ) and thus is strongly shielded. In contrast, after dehydrogenation of 8a via DDQ, the proton H e of 6a is shifted away from the neighboring benzene into its deshielding region, in accordance with a down-field shift of H e in the 1 H NMR spectrum. Moreover, 1 H– 1 H correlation spectroscopy (COSY) and 1 H- 1 H nuclear Overhauser effect spectroscopy (NOESY) analyses (Fig. 3 b, c ) allowed unambiguous assignments of the proton signals of 6a . The structure was further characterized by 1 H– 13 C heteronuclear single-quantum correlation (HSQC) and 1 H– 13 C heteronuclear multiple-bond correlation (HMBC) spectroscopies. The chemical identity of 6a was confirmed by high-resolution matrix-assisted laser desorption/ionization time-of-flight (MALDI-TOF) MS, which showed a matching isotopic pattern starting at m / z = 590.1980, in agreement with the theoretical value of 590.1994 (Fig. 3d ). Fig. 2 Synthesis of diaza-HBP 6a in solution and internally N-doped diaza-HBC 7c upon interfacial confinement. Reagents and conditions: (i) tributylamine, DMSO, 190 °C; (ii) DDQ, C 2 D 2 Cl 4 , 100 °C; (iii) in vacuo on the Ag(111) surface, 270 °C. The calculated nucleus-independent chemical shifts (NICS) values are depicted in blue (unit: ppm), indicating the antiaromatic nature of the pyrazine ring (in parenthesis the NICS(1) value, see text and Supplementary Fig. 1 ) Full size image Fig. 3 Structural characterizations of the in situ generated diaza-HBP 6a . a 1 H NMR spectra of 8a and 6a together with their structural assignments (*C 2 HDCl 4 ). Compared to precursor 8a , the signals of 6a were down-field shifted, corroborating the extension of the π-conjugation. 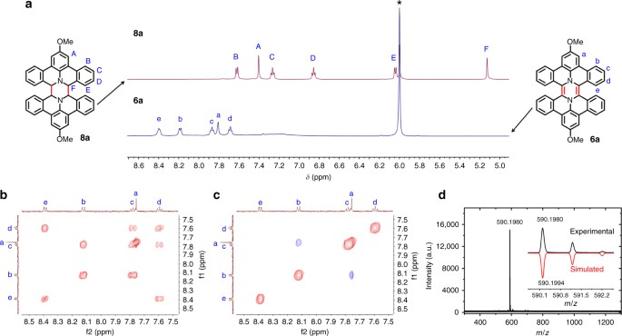Fig. 3 Structural characterizations of the in situ generated diaza-HBP6a.a1H NMR spectra of8aand6atogether with their structural assignments (*C2HDCl4). Compared to precursor8a, the signals of6awere down-field shifted, corroborating the extension of the π-conjugation.bAromatic region of the1H–1H COSY spectrum of6ain C2D2Cl4.cAromatic region of the1H–1H NOESY spectrum of6ain C2D2Cl4.dHigh-resolution MALDI-TOF MS spectrum of6a, with an inset showing its experimental (black line) and simulated isotopic distributions (red line) b Aromatic region of the 1 H– 1 H COSY spectrum of 6a in C 2 D 2 Cl 4 . c Aromatic region of the 1 H– 1 H NOESY spectrum of 6a in C 2 D 2 Cl 4 . d High-resolution MALDI-TOF MS spectrum of 6a , with an inset showing its experimental (black line) and simulated isotopic distributions (red line) Full size image Fig. 4 Photophysical investigations. a Experimental and b TDDFT-simulated absorption spectra of 6a and its precursor 8a . The simulated spectra of 6a showed the appearance of a new band at 577 nm, in accordance with the experimental observation. c X-ray single-crystal structure of 8c . d DFT-optimized structure of 8a . e DFT-optimized structure of 6a Full size image To investigate the photophysical properties of 6a , we prepared diaza-HBP 6a in situ by carrying out the oxidation reaction in a sealed quartz cell and recorded the absorption and photoluminescence spectra. As shown in Fig. 4a , dimer precursor 8a exhibited an absorption maximum at λ max = 390 nm, and an absorption onset at ≈500 nm. After dehydrogenation, the absorption maximum barely changed, but a new band emerged in the range of 500 to 630 nm, suggesting an extended π-conjugation. To further understand the photophysical properties, DFT calculations were performed on both 8a and 6a . In order to determine the exact molecular geometry of 8a , growth of single crystals of 8a–c was pursued and a single crystal of 8c suitable for X-ray analysis was successfully obtained, revealing an anti -folded structure (Fig. 4c ). Thus, the anti -folded geometry was employed as input geometry for the DFT optimization of similar precursors (Fig. 4d ). DFT studies on dehydrogenated 6a indicate that the anti -folded conformation (Fig. 4e ) is energetically preferred compared to the twisted one. Time-dependent DFT (TDDFT) calculations of 6a and 8a indicated that the emerging absorption band of 6a can be attributed to the HOMO→LUMO + 2 transition (Fig. 4b and Supplementary Tables 1 – 3 ). The HOMO→LUMO transition of 6a is symmetry forbidden, and 6a is non-emissive, in agreement with previous reports on antiaromatic systems [32] , [33] . On-surface synthesis of 7c Despite generation of diaza-HBP 6a through solution synthesis, further characterization of 6a was restricted by its low stability. In addition, attempts to oxidize intermediate product 8a–c directly to diaza-HBC derivatives resulted in insoluble solids, which could not be characterized. This led us to adapt the solution chemistry of PAMYs to on-surface synthesis [34] , [35] , [36] , [37] , which offers today a new approach to organic chemistry. We thus deposited 5c on Ag(111) by molecular beam evaporation (Methods section and Supplementary Fig. 2 ). Upon annealing to 270 °C, small quantities of diaza-HBC 7c were detected as displayed in Fig. 5a . Unlike solution synthesis (Fig. 2 ), no intermediate product 8c was identified after annealing the deposited 5c in several ultra-high vacuum (UHV) preparations on Ag(111), Ag(100), Cu(111), and boron nitride (BN) on Cu(111), suggesting that homocoupling and dehydrogenation occur synergistically at the employed reaction temperatures. Notably, 7c was detected on BN/Cu(111) templates [38] at similar annealing temperatures in trace-quantities (Supplementary Fig. 3 ), indicating that the on-surface coupling strategy proceeds in a metal-free fashion, further motivating studies on reaction mechanisms and on-surface synthesis on insulators. Fig. 5 On-surface homocoupling of precursor 5c yields fully planar and neutral diaza-HBC 7c on Ag(111). a Scanning tunneling microscopy (STM) overview of reaction product and unreacted species on Ag(111). V s = 30 mV, I t = 10 pA. b Constant-height STM data of diaza-HBC with partially superposed molecular model. V s = 5 mV. c Frequency-modulated atomic force microscopy (FM-AFM) and d Laplace-filtered FM-AFM data reveal details in the molecular structure. Apparent C = C distance 1.0 Å (black), and N–C 1.8 Å (blue). e FM-AFM simulations of 7c employing a neutral tip. Apparent C = C distance 1.5 Å (black), N–C 1.5 Å (blue). f FM-AFM simulations employing a negatively charged probe tip. Apparent C = C distance 1.3 Å (black), N-C 1.9 Å (blue). For simulation parameters see Methods. g – n Constant-height STM data ( g , i , k , m ) at different biases and corresponding ( h , j , l , n ) DFT simulations. White arrows point to N atoms oriented along the diaza-HBC symmetry axis. Scale bars ( a ) 20 Å, ( b – f ) 2 Å, ( g – n ) 5 Å Full size image High-resolution, constant height STM (Fig. 5b ) and FM-AFM (Fig. 5c, d ), using CO-functionalized tips, confirmed 7c on Ag(111). In FM-AFM data on Ag(111), the central pyrazine ring of 7c (Fig. 5d ) appears distorted. Observation of a D 2 h symmetry points toward the nitrogen atoms sitting at the positions indicated by white arrows. Note that the predicted DFT C=C bond length of the central pyrazine ring is 1.40 Å vs. 1.42 Å for the N–C bond, and the molecule remains planar (z ± 0.05 Å) for calculated adsorption sites on Ag(111) (Supplementary Fig. 4 ). Bond lengths in AFM data typically undergo distorsions [27] , [39] , [40] , [41] especially under the influence of electrostatic interactions with the CO tip [42] , [43] , [44] , [45] , [46] . This causes a distorted appearance of the central pyrazine ring. Quantitative evidence of these combined effects is summarized in the AFM frequency shift simulation including a DFT-derived electrostatic potential (Fig. 5e, f, see Methods section). Note how the apparent C=C bond length in the simulated image (1.3 Å) appears shorter than the apparent N–C bond length (1.9 Å, Fig. 5f ), in good agreement with the experimental data (1.0 and 1.8 Å, respectively). When a neutral tip is employed for the AFM simulation the central pyrazine ring is fully symmetric, with apparent N–C and C=C lengths of 1.5 Å (Fig. 5e ), confirming that the distortions in the FM-AFM data originate mostly from electrostatic effects. Combined scanning probe data and theoretical investigations indicate that 7c remains neutral (conserving its pyrazine 8π state) on the surface, which is a requirement for antiaromaticity. 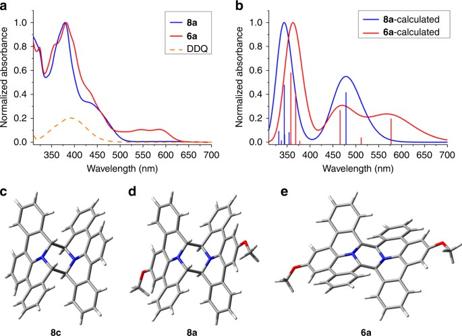Fig. 4 Photophysical investigations.aExperimental andbTDDFT-simulated absorption spectra of6aand its precursor8a. The simulated spectra of6ashowed the appearance of a new band at 577 nm, in accordance with the experimental observation.cX-ray single-crystal structure of8c.dDFT-optimized structure of8a.eDFT-optimized structure of6a Bader charge analysis was employed to assess molecule-substrate charge transfer. As shown by NICS calculations on isolated molecules, a neutral species of 7c implies an 8π pyrazine unit, which is antiaromatic in the isolated state. 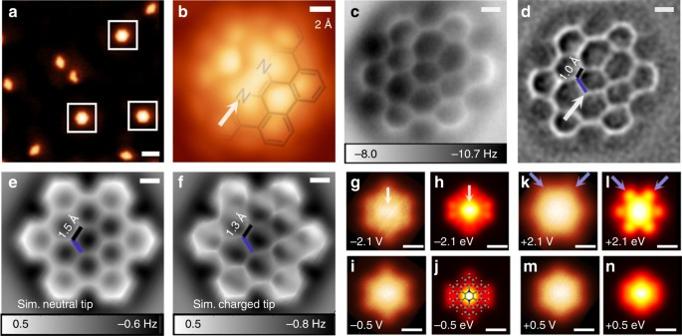Fig. 5 On-surface homocoupling of precursor5cyields fully planar and neutral diaza-HBC7con Ag(111).aScanning tunneling microscopy (STM) overview of reaction product and unreacted species on Ag(111).Vs= 30 mV,It= 10 pA.bConstant-height STM data of diaza-HBC with partially superposed molecular model.Vs= 5 mV.cFrequency-modulated atomic force microscopy (FM-AFM) anddLaplace-filtered FM-AFM data reveal details in the molecular structure. Apparent C = C distance 1.0 Å (black), and N–C 1.8 Å (blue).eFM-AFM simulations of7cemployinganeutral tip. Apparent C = C distance 1.5 Å (black), N–C 1.5 Å (blue).fFM-AFM simulations employing a negatively charged probe tip. Apparent C = C distance 1.3 Å (black), N-C 1.9 Å (blue). For simulation parameters see Methods.g–nConstant-height STM data (g,i,k,m) at different biases and corresponding (h,j,l,n) DFT simulations. White arrows point to N atoms oriented along the diaza-HBC symmetry axis. Scale bars (a) 20 Å, (b–f) 2 Å, (g–n) 5 Å Upon oxidation, a positively charged “7π” radical cation state of the diaza-HBC 7c displays significantly reduced antiaromaticity and a “6π” dication species exhibits an aromatic character (Supplementary Fig. 1 ). On Ag(111), theoretical charge analysis finds only marginal electron transfer to the substrate (the molecule is charged positively by less than + 0.14 e for all calculated molecular configurations on Ag(111), Supplementary Fig. 4 ). Moreover, when trying to enforce molecular charging by removing electrons from the calculated system, the charge at the molecule was only increased to about + 0.8 e , when the whole 29 Å × 25 Å × 22 Å unit cell was charged by + 10 e . These theoretical analyses indicate that 7c remains in the neutral “8π” state on Ag(111). The good correlation of the STM experimental data with Tersoff-Hamann simulations supports the validity of the theoretical conclusions (Fig. 5g, n and see Supplementary Fig. 5 for extended comparisons). It should be noted how at negative energies (voltages), the symmetry of the tunneling image follows the diaza-HBC 7c hexagonal frame (marked by a white arrow, Fig. 5g, h ). At high positive biases (between 0.9 and 2.1 eV, see Supplementary Fig. 5 ) the symmetry of the tunneling data is rotated (blue arrows, Fig. 5k, l ) with respect to the diaza-HBC hexagonal frame, that is, tunneling is enhanced between the bay regions in the periphery of diaza-HBC. Notably, between −0.5 and 0.5 eV (Fig. 5i, j, m, n ), both experiment and simulation follow the hexagonal symmetry of 7c on Ag(111). Having identified a neutral state of 7c on Ag(111), comparison between 7c on Ag(111) and the isolated antiaromatic species provides evidence on the preserved antiaromatic character of 7c on Ag(111). 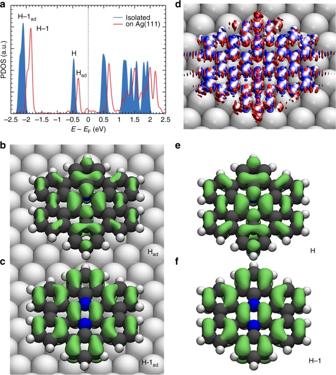Fig. 6 DFT electronic structure comparison of the isolated and Ag(111)-supported diaza-HBC7c.aProjectedpzcontributions to the density of states of isolated7c(blue) and on Ag(111). The Fermi energy (EF) of the isolated molecule has been arbitrarily defined for comparison.b,cContribution of the highest occupied molecular orbitalHad(at −0.32 eV ina) and (H-1)adto7con Ag(111).dElectron density difference between7con Ag(111) and the isolated molecule plus isolated substrate. Red regions represent electron density depletion, whilst blue electron density gain. Atoms are rendered translucent.e,fHighest occupied molecular orbitalHandH-1of isolated7c. These results suggest that antiaromatic character is preserved on Ag(111) Figure 6 depicts the site-projected density of states (PDOS) as well as plots for the individual Kohn-Sham orbitals. Only marginal hybridization resulting in mid-gap states is observed when the isolated molecule interacts with Ag(111) (Fig. 6a , red line). The mid-gap states do not appear to significantly influence the antiaromatic character of the adsorbed molecule: the HOMO (H) and HOMO-1 (H-1) signatures of isolated 7c are reflected undisturbed at the surface (compare Fig. 4 b, c, e, f). Instead, the electronic density difference plot (Fig. 6d ) shows that the mid-gap states originate from homogeneous orbital contributions, including the role of rings which are considered to be aromatic (Supplementary Fig. 1 ). Note that scanning tunneling spectroscopy follows the major theoretical LDOS features including a pronounced broadening (Supplementary Fig. 6 ). Fig. 6 DFT electronic structure comparison of the isolated and Ag(111)-supported diaza-HBC 7c . a Projected p z contributions to the density of states of isolated 7c (blue) and on Ag(111). The Fermi energy ( E F ) of the isolated molecule has been arbitrarily defined for comparison. b , c Contribution of the highest occupied molecular orbital H ad (at −0.32 eV in a ) and ( H-1 ) ad to 7c on Ag(111). d Electron density difference between 7c on Ag(111) and the isolated molecule plus isolated substrate. Red regions represent electron density depletion, whilst blue electron density gain. Atoms are rendered translucent. e , f Highest occupied molecular orbital H and H-1 of isolated 7c . These results suggest that antiaromatic character is preserved on Ag(111) Full size image In summary, we have demonstrated the chemical synthesis of a partially fused PAH in solution and the on-surface synthesis of a fully planarized nanographene molecule with antiaromatic pyrazine dopants. Diaza-HBP 6a has been achieved in solution and investigated by NMR, high-resolution MALDI-TOF MS and UV-vis absorption spectroscopy, while the fully cyclized diaza-HBC 7c has been successfully fabricated on Ag(111) and characterized by STM and FM-AFM. We suggest that pyrazine rings are potential candidates to be included in 2D materials to spawn novel functional properties induced by breaking the conjugated lattice via antiaromatic ring dopants. Importantly, the chemistry of on-surface azomethine ylide homocoupling reported here opens up a new route to novel nanographene materials, especially graphene nanoribbons, on a large variety of substrates. Procedure for the in situ preparation of 6a Inside an argon-filled glovebox, precursor 8a (2.0 mg, 1.0 eq. ), DDQ (15 mg, 20 eq.) and C 2 D 2 Cl 4 (0.6 mL) were added sequentially into a sealable NMR tube. The mixture was heated at 100 °C for 1 min and cooled down to room temperature, and then analyzed by NMR spectroscopy. Synthetic procedures and characterization data of 8a–c and 6a are provided in the Supplementary Methods and Supplementary Figs. 7 – 45 . STM and FM-AFM measurements Precursor 5c was sublimated between 200 °C and 220 °C at 10 −9 mbar. Data was acquired in situ using a CreaTec STM/AFM (5.5 K) under ultra-high vacuum (10 −10 mbar). AFM data were taken in constant height mode at 0.0 V bias, using a qPlus sensor (resonance frequency ≈22 kHz, oscillation amplitude: 70 pm to 100 pm). The tungsten tip was prepared by focused-ion beam processing and in situ tip forming. For subsequent tip functionalization, carbon monoxide (CO) was dosed on the cold sample and transferred to the tip. The images were processed using the Gwyddion software package [47] . Computational details DFT Calculations in Fig. 4 were performed using the Gaussian 09 software package. The geometries were optimized at the B3LYP/6-311 G(d,p) level. The excitation energies were calculated by the TDDFT method at the B3LYP/6-311 G(d,p) level. NICS were calculated using the gauge invariant atomic orbital (GIAO) approach at the GIAO-B3LYP/6-311 + G(2d,p) level. NICS(1) values were averaged by two positions (above and below the plane). For Figs. 5 and 6 , periodic DFT calculations were performed with the VASP code [48] , projector augmented wave potentials [49] and plane waves expanded to a kinetic energy cutoff of 400 eV. Exchange-correlation effects were treated by the van der Waals density functional [50] in the version denoted as rev-vdWDF2 [51] . The Ag(111) surface was represented by four layered slab separated by approx. 15 Å of vacuum region. Furthermore, a p (10×10) super cell was used together with a 2×2 k -point sampling. All structures were geometrically optimized until the residual forces on all atoms were smaller than 0.01 eV/Å, except for the bottom two layers of the slab, which were frozen in the bulk distance. An exhaustive conformational search identified the preferred adsorption site (Site b, Supplementary Fig. 4 ). The site’s adsorption height was further optimized for a gas-phase molecule and found to be 3.22 Å between the molecular and metallic planes (Site c, Supplementary Fig. 4 ). This site was employed to simulate the STM and AFM images. STM images were simulated with the Tersoff-Hamann approximation [52] using the implementation by Lorente and Persson [53] . AFM simulations were performed with a modification of the particle probe model code [42] by Hapala et al. The DFT-derived Hartree potential was employed to prepare an electrostatic grid which together with the molecular Lennard-Jones potential acted as the force-field for simulating the frequency shift of a probe C = O particle as detailed in ref. [46] . The simulations involved oscillating a probe particle with an amplitude of 5 Å at a height of 7.7 Å above the substrate. The terminal oxygen was given a negative charge of - 0.005 e . The probe’s stiffness x,y,z components were set to 3 N m −1 , 3 N m −1 and 50 N m −1 , respectively. Data availability X-Ray crystallographic data can be obtained free of charge from the Cambridge Crystallographic Data Centre (CCDC) with the CCDC number 1529624 via its website ( https://www.ccdc.cam.ac.uk/structures/ ). All other data are available within the article and its Supplementary Information or from the corresponding authors upon reasonable request.